Optical visualization of individual ultralong carbon nanotubes by chemical vapour deposition of titanium dioxide nanoparticles Direct visualization and manipulation of individual carbon nanotubes in ambient conditions is of great significance for their characterizations and applications. However, the observation of individual carbon nanotubes usually requires electron microscopes under high vacuum. Optical microscopes are much more convenient to be used, yet their resolution is low. Here we realize the visualization and manipulation of individual ultralong carbon nanotubes under optical microscopes by deposition of TiO 2 nanoparticles on them. The strong scattering of TiO 2 nanoparticles to visible light renders them visible by optical microscopes. Micro-Raman-spectroscopy measurement of individual carbon nanotubes is greatly facilitated by their optical visualization. With the assistance of TiO 2 nanoparticles, individual carbon nanotubes can be easily manipulated under an optical microscope at macroscopic scale and in ambient conditions. Based on our approach, various manipulation of ultralong carbon nanotubes, including cutting, transfer, fabrication of structures/devices and pulling out inner shells of multiwalled carbon nanotubes, are demonstrated. The advance of material science always benefits from the development of modern characterization or operation techniques. Carbon nanotubes (CNTs) are undoubtedly one of the most attractive materials in the past two decades because of their superior properties and potential applications in many fields. Particularly, ultralong CNTs, with their perfect one-dimensional nanostructures and excellent properties, such as extraordinary mechanical strength, ultrahigh electron mobility and excellent electrical conductivity [1] , [2] , [3] , are promising building blocks for high-performance fibres and nanodevices. However, the direct visualization, location and manipulation of individual CNTs, especially single or few-walled CNTs, is extremely difficult because of their nanosized diameters. Advanced analytical equipment, such as scanning electron microscope (SEM), transmission electron microscope (TEM) and atomic force microscope (AFM) and so on, has been employed to characterize the location, morphology and structure of CNTs. The in-situ manipulation of individual CNTs with the help of the above equipment has also been realized [4] , [5] , [6] , [7] , [8] . However, all the above-mentioned techniques cannot guarantee the efficient location and manipulation of ultralong CNTs, because of their characteristics such as limited accessibility, requiring high vacuum, narrow field of view and/or small operating space. Optical microscopes are routine facilities in many laboratories. Combing with the open-operation space of optical microscopes, if individual CNTs can be directly observed with an optical microscope, the in-situ observation and manipulation of ultralong CNTs will become much easier. However, the resolution of optical microscopes is much lower than that of SEM, TEM and AFM. Recently, various methods were proposed to ‘see’ CNTs optically, such as near-field Raman spectroscopy [9] and fluorescence microscopy [10] , [11] , [12] , [13] , [14] . However, the preparation of the samples and the identification of individual CNTs are quite complex and time-consuming by these techniques. Besides, an electro-deposition process of Ag nanoparticles (NPs) [15] and a seeded electroless deposition process of Au NPs [16] have been used to visualize individual CNTs on substrates under an optical microscope. Compared with CNTs sitting on substrates, suspended CNTs possess the pristine properties of CNTs and are convenient to be manipulated. However, the above strategies cannot be applied on suspended CNTs because of the fact that these processes are conducted in liquid phases that will destroy the suspended CNTs. Therefore, to explore the full potential of CNTs towards their future applications, a facile and nondestructive visualization method for individual suspended CNTs, especially for those with length up to several centimeters, is in great demand. In this contribution, a facile and effective method to visualize individual suspended ultralong CNTs by deposition of TiO 2 NPs in a vapour phase is proposed. The strong scattering of TiO 2 NPs to visible light enables the CNTs to be easily observed under optical microscopes even at low magnification, which allows the direct manipulation of individual CNTs, even ultralong ones with length up to centimeters, under optical microscopes. Based on that, we demonstrate various manipulations of individual ultralong CNTs under an optical microscope. Deposition of TiO 2 NPs on individual ultralong CNTs The process of depositing TiO 2 NPs on ultralong CNTs is illustrated in Fig. 1a–d and Supplementary Fig. S1 . Suspended ultralong CNTs were grown by chemical vapour deposition [1] , [17] , [18] on a silicon substrate containing many trenches (0.5–1 mm in width and 0.5 mm in depth). The as-grown CNTs were brought into contact with TiCl 4 vapour for in-situ deposition of TiO 2 NPs (see Methods section for details). 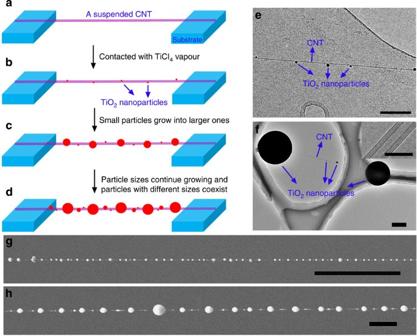Figure 1: Deposition of TiO2NPs on ultralong CNTs. (a–d) Schematic illustration for depositing TiO2NPs on suspended CNTs. (e) TEM images of CNTs with small TiO2NPs prepared with contact time of 0.1–0.3 s. Scale bar, 200 nm. (f) TEM image of CNT with TiO2NPs with various sizes prepared with contact time of 7.0 s. Scale bar, 500 nm. Inset: high-resolution TEM image of the CNT shown in panelf. Scale bar, 5 nm. (g,h) SEM images of suspended CNTs decorated with TiO2NPs prepared with contact time of 5.0 s. Scale bar, 10 μm (ing); 2 μm (inh). Figure 1: Deposition of TiO 2 NPs on ultralong CNTs. ( a – d ) Schematic illustration for depositing TiO 2 NPs on suspended CNTs. ( e ) TEM images of CNTs with small TiO 2 NPs prepared with contact time of 0.1–0.3 s. Scale bar, 200 nm. ( f ) TEM image of CNT with TiO 2 NPs with various sizes prepared with contact time of 7.0 s. Scale bar, 500 nm. Inset: high-resolution TEM image of the CNT shown in panel f . Scale bar, 5 nm. ( g , h ) SEM images of suspended CNTs decorated with TiO 2 NPs prepared with contact time of 5.0 s. Scale bar, 10 μm (in g ); 2 μm (in h ). Full size image After the suspended CNTs contacted TiCl 4 for 1–7 s, many TiO 2 NPs deposited on the CNTs. Figure 1e–h show the necklace-like CNT TiO 2 hybrids. Most of the large TiO 2 NPs have spheric morphologies with diameters of 100–1,000 nm. Most of these spherical TiO 2 NPs completely wrap the suspended CNTs, forming coaxial structures ( Fig. 1f–h ). In contrast, other particles, especially those with small diameters (20–100 nm), usually adhere to the outer wall of suspended CNTs ( Fig. 1e ). Small TiO 2 NPs are distributed between adjacent large TiO 2 NPs. The interspace of the small NPs usually ranges from 20 to 1000, nm, whereas the interspace of larger NPs usually ranges from 1 to 5 μm. Pristine CNT segments can be clearly observed between the particles. The ultralong CNT shown in Fig. 1f is a triple-walled CNT with a diameter of 3.5 nm (see the inset in Fig. 1f ). Compared with the depostion methods of TiO 2 NPs on CNTs reported previously [19] , [20] , [21] , [22] , [23] , [24] , [25] , the vapour phase-directed deposition reported here is easy to be conducted and does not require the CNT surfaces to be pre-modified. Although a series of covalent and non-covalent methods have been reported to deposit metal [26] , [27] , [28] , [29] , [30] or metal oxide NPs [19] , [20] , [21] , [22] , [23] , [24] , [25] , [30] , [31] , [32] , [33] , [34] , [35] , [36] , [37] , [38] , [39] , [40] , [41] , [42] on CNTs, most of these methods require the CNTs to be functionalized or modified with surfactants [39] , [42] , and the processes are conducted in liquid phases [17] , [18] , [19] , [20] , [21] , [22] , [23] , [24] , [25] , [26] , [27] , [28] , [29] , [30] , [31] , [32] , [33] , [34] , [35] , [36] , [37] , [38] , [39] , [41] , [42] . These strategies cannot be applied on individual suspended ultralong CNTs because of the fact that they will destroy the suspended CNTs. Besides, atomic layer deposition [43] , which avoids the use of liquid phases, has been used to conformably coat CNTs sitting on substrates [41] , [43] or pre-functionalized suspended CNTs [44] with metal oxide films. In comparison, we realized the deposition of TiO 2 NPs on as-prepared suspended CNTs in a vapour phase. TiCl 4 , which is a highly volatile metal halide, was used as the precusor for TiO 2 NPs. TiCl 4 forms misty smog of TiO 2 and HCl upon contact with humid air [45] . When TiCl 4 vapour gets into contact with suspended CNTs, tiny TiO 2 NPs nucleate on the CNTs ( Fig. 1b ). The suspended CNTs have a role of templates in tailoring the size of TiO 2 NPs [35] . The TiO 2 NPs are hydrophilic [46] , whereas the pristine CNTs are hydrophobic [47] . As a result, the following formed TiO 2 in the vapour phase prefers to deposite on the preformed TiO 2 nucleus. The −OH groups on the surface of TiO 2 NPs also catalyse TiCl 4 hydrolysis [48] , resulting in the vapour phase epitaxial growth of the preformed TiO 2 NPs. The small TiO 2 NPs attached on the outer wall of the suspended CNTs gradually grow large and wrap the CNTs with the continuously growth, forming coaxial strucutures. Meanwhile, a large amount of newly nucleated TiO 2 NPs formed and adhered to the suspended CNTs. Therefore, small and large TiO 2 NPs coexist on the suspended CNTs. The interactions between the TiO 2 NPs and the CNTs is dominated by van der Waals force [22] , [35] . The contact time of CNTs with the TiCl 4 vapour and the air humidity have important roles in determining the diameter and number distribution of the TiO 2 NPs deposited on the suspended CNTs as reported previously [22] . As shown in Supplementary Fig. S2 , the diameter and number of the TiO 2 NPs are proportional with the contact time and the relative air humidity. The size of the TiO 2 NPs on CNTs obeys a typical logarithmic normal distribution as shown in Supplementary Fig. S2a . Supplementary Table S1 shows the diameter and interspace distribution of TiO 2 NPs with different contact time. With the increase of contact time, the mean diameter of TiO 2 NPs ( μ ) increases, whereas the particle interspace decreases ( Supplementary Fig. S2b ). No matter what the interspace is, the variance of the interspace is <0.1 μm 2 , indicating that the interspace of the TiO 2 NPs is uniform. The air humidity affects the hydrolysis rate of TiCl 4 . The higher the air humidity, the larger the hydrolysis rate is. As a result, μ increases with the increase of air humidity ( Supplementary Fig. S2c ). When the relative air humidity is >70%, the increasing trend of μ gradually slows down because of the hydrolysis rate reaching its limit. Optical visualization of individual ultralong CNTs The diameters of most TiO 2 NPs (100–1,000 nm) are comparative with the wavelength of visible light (300–700 nm), rendering the TiO 2 NPs a strong Mie-scattering ability [49] , [50] , [51] . The CNTs decorated with TiO 2 NPs can be easily observed and tracked under an optical microscope. 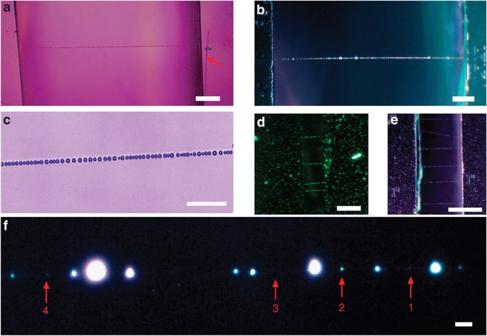Figure 2: Optical images of suspended CNTs. (a,c) Bright field modes. The red arrow in panelashows a broken CNT falling on the substrate. Scale bar, 100 μm (ina); 20 μm (inc). (b) Dark field mode. Scale bar, 100 μm. (d,e) Optical images with low magnification (× 50). Scale bar, 1 mm. The light source in paneldis green laser, whereas the light source in paneleis visible light. (f) High-resolution optical image of a suspended CNT decorated with TiO2NPs. The small TiO2NPs indicated by the red arrows have diameters <200 nm. Scale bar, 1 μm. Figure 2 shows typical optical images of suspended CNTs decorated with TiO 2 NPs. We can easily locate and track the suspended CNTs with the aid of TiO 2 NPs. Even when the suspended CNTs with TiO 2 NPs are broken and finally fall down onto the substrate, they can still be clearly observed (shown by the red arrow in Fig. 2a ). No matter for what incident light intensity, the TiO 2 NPs always have a strong scattering ability to the incident light ( Fig. 2a–c ), especially in the dark field mode ( Fig. 2b ). The suspended CNTs decorated with TiO 2 NPs can be clearly observed even with a very low magnification (× 50) of microscopes ( Fig. 2d ). Particularly, TiO 2 NPs as small as 100 nm ( Fig. 2f , shown by arrow ‘3’) are still visible under the optical microscope. Furthermore, the TiO 2 NPs can be removed through an acid-washing method to facilate their futher characterizations and applications ( Supplementary Fig. S3 ). Figure 2: Optical images of suspended CNTs. ( a , c ) Bright field modes. The red arrow in panel a shows a broken CNT falling on the substrate. Scale bar, 100 μm (in a ); 20 μm (in c ). ( b ) Dark field mode. Scale bar, 100 μm. ( d , e ) Optical images with low magnification (× 50). Scale bar, 1 mm. The light source in panel d is green laser, whereas the light source in panel e is visible light. ( f ) High-resolution optical image of a suspended CNT decorated with TiO 2 NPs. The small TiO 2 NPs indicated by the red arrows have diameters <200 nm. Scale bar, 1 μm. Full size image Micro-Raman spectra measurement of individual CNTs is greatly facilitated by the optical visualization of individual CNTs. With the assistance of TiO 2 NPs, the position and orientation of the ultralong suspended CNTs can be easily identified under the optical microscope of micro-Raman-spectroscopy equipment. The laser spot can be focused on the pristine CNTs between two adjacent TiO 2 NPs ( Fig. 3a ), where strong Raman scattering signals are usually obtained. The deposition of TiO 2 NPs does not influence the Raman spectra of CNTs. 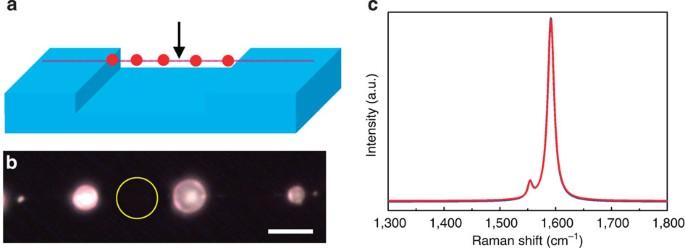Figure 3: TiO2NP-assisted micro-Raman spectra measurement of a suspended CNT. (a) Illustration for micro-Raman spectra measurement. (b) Optical image showing the position of laser spot (yellow circle) on the suspended CNTs for micro-Raman spectra measurement. Scale bar, 1 μm. (c) Raman spectra of the same CNT before (the red line) and after (the blue line) deposition of TiO2NPs. Figure 3c shows the Raman G-band of a CNT before and after deposition of TiO 2 NPs. The Raman spectra measured with and without TiO 2 NPs were almost the same (see Supplementary Discussion and Supplementary Fig. S4 ). Figure 3: TiO 2 NP-assisted micro-Raman spectra measurement of a suspended CNT. ( a ) Illustration for micro-Raman spectra measurement. ( b ) Optical image showing the position of laser spot (yellow circle) on the suspended CNTs for micro-Raman spectra measurement. Scale bar, 1 μm. ( c ) Raman spectra of the same CNT before (the red line) and after (the blue line) deposition of TiO 2 NPs. Full size image Furthermore, the visualization of individual CNTs under optical microscopes enabled by the deposition of TiO 2 NPs greatly facilitates the manipulation of individual CNTs in macro scale and ambient conditions. For example, with the assistance of TiO 2 NPs, ultralong CNTs can be cut and the as-obtained CNT segments can be used as samples for further characterization. 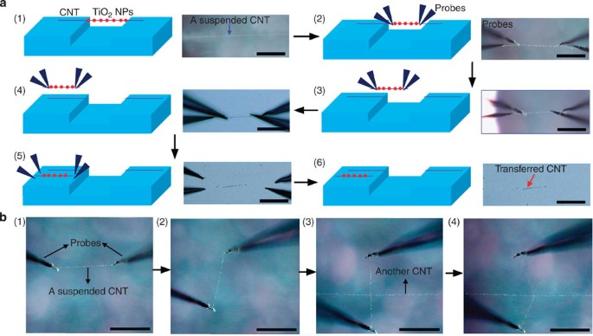Figure 4: Cutting and transferring of individual CNTs and fabrication of a CNT cross-structure. (a) Cutting and transferring of individual CNTs (left: schematic illustration; right: optical images). (1) A suspended CNT with TiO2NPs. Scale bar, 50 μm. (2) Four probes were moved onto the CNT to cut a CNT segment. Scale bar, 50 μm. (3–6) A CNT segment (ca. 70 μm) was cut off from the CNT. Scale bar, 50 μm. Then the probes served as tweezers to transfer the CNT segment. (b) Cutting a CNT segment and fabricating a CNT cross-structure. (1) Cutting a CNT segment from a suspended CNT using two probes. Scale bar, 50 μm. (2) Changing the position and orientation of the CNT segment. Scale bar, 50 μm. (3) Moving the CNT segment onto another CNT and fabricating a CNT cross-structure. Scale bar, 50 μm. (4) Deforming the CNT cross-structure by moving the probes. Scale bar, 50 μm. Figure 4a shows a process of cutting and transferring a CNT segment. The cut-off CNT segments can be used for structural or property measurements, such as micro-Raman spectra measurement, TEM characterization and electrical measurement, facilitating the characterization of ultralong CNTs. Moreover, the CNT segments can be employed to fabricate complicated CNT architectures. Figure 4b shows a process to fabricate a CNT cross-structure, which can be completed within several minutes. More complicated CNT architectures could be fabricated in the same way. Note that all the above procedures were carried out under an optical microscope, which provides an open space for the manipulation of individual CNTs. Figure 4: Cutting and transferring of individual CNTs and fabrication of a CNT cross-structure. ( a ) Cutting and transferring of individual CNTs (left: schematic illustration; right: optical images). (1) A suspended CNT with TiO 2 NPs. Scale bar, 50 μm. (2) Four probes were moved onto the CNT to cut a CNT segment. Scale bar, 50 μm. (3–6) A CNT segment (ca. 70 μm) was cut off from the CNT. Scale bar, 50 μm. Then the probes served as tweezers to transfer the CNT segment. ( b ) Cutting a CNT segment and fabricating a CNT cross-structure. (1) Cutting a CNT segment from a suspended CNT using two probes. Scale bar, 50 μm. (2) Changing the position and orientation of the CNT segment. Scale bar, 50 μm. (3) Moving the CNT segment onto another CNT and fabricating a CNT cross-structure. Scale bar, 50 μm. (4) Deforming the CNT cross-structure by moving the probes. Scale bar, 50 μm. Full size image The optical visualization of individual CNTs also facilitates the design and fabrication of various devices. Figures 5a show that a suspended CNT can be bent by a gas flow, which can be used to monitor external gas flows. Accordingly, given a known gas velocity, this phenomenon can be used to measure the tensile strength and Young’s modulus of the suspended CNTs. 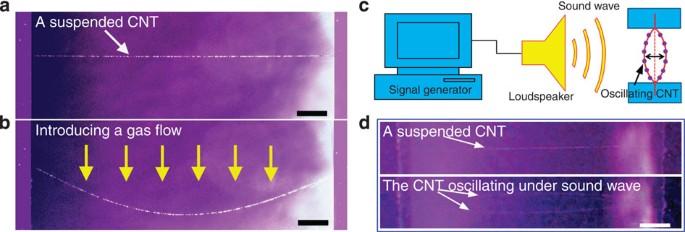Figure 5: Gas-flow-induced bending and sound-wave-induced oscillation of suspended CNTs. (a) A suspended CNT. Scale bar, 100 μm. (b) Gas-flow-induced bending of the CNT. Scale bar, 100 μm. (c) Illustration of oscillating a suspended CNT with sound wave. (d) Snapshot images of an oscillating CNT under sound wave. Scale bar, 100 μm. Figure 5c show that a suspended CNT/TiO 2 chain oscillates under a sound wave, which can be monitored by an optical microscope. This phenomenon can be used to test the fatigue life of the suspended CNTs. Besides, an external electric field can also be used to manipulate suspended CNT/TiO 2 chain, exhibiting interesting behaviours ( Supplementary Fig. S5 ). Similarly, more devices based on individual CNTs could be fabricated and more properties of individual CNTs could be measured with the TiO 2 NP-assisted optical visualization of CNTs. Figure 5: Gas-flow-induced bending and sound-wave-induced oscillation of suspended CNTs. ( a ) A suspended CNT. Scale bar, 100 μm. ( b ) Gas-flow-induced bending of the CNT. Scale bar, 100 μm. ( c ) Illustration of oscillating a suspended CNT with sound wave. ( d ) Snapshot images of an oscillating CNT under sound wave. Scale bar, 100 μm. Full size image Moreover, with the aid of TiO 2 NPs, the intershell sliding behaviours of ultralong multiwalled CNTs can be tracked and investigated in macroscopic scale under an optical microscope. 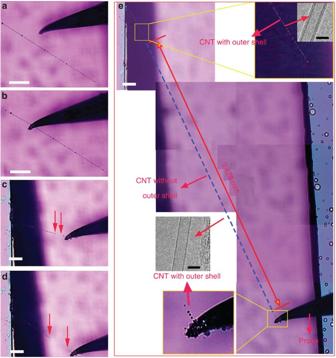Figure 6: Pulling out the inner tube from a DWCNT. (a,b) Approaching a probe to a DWCNT and then contacting it. Scale bar, 100 μm. (c,d) Stretching the DWCNT and then pulling out its inner shell. Scale bar, 200 μm. (e) A 3.43-mm-long singlewalled CNT being pulled out from the DWCNT. Scale bar, 20 μm; 2 nm (lower inset); 2 nm (upper inset). Figure 6a shows a suspended double-walled CNT (DWCNT) (see its high-resolution TEM image in the upper inset in Fig. 6e ) and a probe for manipulation. With the probe approaching and finally contacting with the CNT, the CNT firmly fixed to the probe due to the strong van der Waals force between them ( Fig. 6b ) (binders such as silver paste could be used for a better fixation effect). Then, the suspended CNT could be stretched by moving the probe in a certain direction. The TiO 2 NPs deposited on the suspended CNT are excellent markers to locate the outer shell of the CNT. During the process, the interspace of two adjacent NPs (shown by two red arrows in Fig. 6c ) suddenly had an increase, indicating that the outer shell of the DWCNT was broken. Although the pulled-out inner shell could not be observed directly under an optical microscope, its location and length could be determined from the broken ends of the outer shell. Figure 6d–e shows that the inner shell of the suspended DWCNT had been continuously pulled out, resulting in a 3.43-mm-long singlewalled CNT. Note that this is the longest inner tube pulled out from a multiwalled CNT, at least two orders of magnitude longer than that of previous reported results [52] . Moreover, if we fix a force cantilever onto the probe, the external force needed for pulling out the inner shell of the CNT and the friction between shells of the CNT could be measured. The tensile strength, breaking strain of the CNTs, could also be obtained. Figure 6: Pulling out the inner tube from a DWCNT. ( a , b ) Approaching a probe to a DWCNT and then contacting it. Scale bar, 100 μm. ( c , d ) Stretching the DWCNT and then pulling out its inner shell. Scale bar, 200 μm. ( e ) A 3.43-mm-long singlewalled CNT being pulled out from the DWCNT. Scale bar, 20 μm; 2 nm (lower inset); 2 nm (upper inset). Full size image In conclusion, the optical visualization of individual CNTs was realized by deposition of TiO 2 NPs on suspended ultralong CNTs in a vapour phase. TiO 2 NPs were uniformly deposited on suspended CNTs using TiCl 4 as the precursor, forming necklace-like CNT TiO 2 hybrids. With the strong scattering to visible light, the TiO 2 NPs could be easily observed under optical microscopes, enabling the facile location and tracking individual CNTs. Mico-Raman spectra measurement was greatly facilitated by the optical visualization of individual CNTs. Besides, with the assistance of TiO 2 NPs, direct manipulation of individual ultralong CNTs in macro scale and under ambient conditions could be easily carried out. We showed that, individual CNTs could be cut, transferred and fabricated into structures/devices. Moreover, we demonstrated the pulling out of an inner shell with a length up to 3.43 mm from a DWCNT under an optical microscope. Our results indicate that the TiO 2 NP-assisted optical visualization of individual CNTs greatly facilitates the characterization and manipulation of individual CNTs, and opens opportunities to explore macro-scale properties of individual CNTs. Note that the NP-assisted optical visualization of CNTs could be easily applied on other nanomaterials, especially one-dimensional, suspended ones. More studies related to the macro-scale mechanical properties of individual ultralong CNTs based on this technique are under way in our laboratory. Deposition of TiO 2 NPs on CNTs The deposition process was conducted at room temperature in a fume hood, where there was a humidity controller to regulate and measure the relative air humidity ( Supplementary Fig. S1 ). TiCl 4 liquid was controllably introduced into a beaker. The TiCl 4 liquid immediately formed misty smog of TiO 2 and HCl upon contact with humid air. The substrates with suspended CNTs were taken into contact with TiCl 4 vapour and TiO 2 smog for deposition of TiO 2 NPs. The contact time usually ranged from 3.0 to 7.0 s. After that, the substrates with suspended CNTs were taken away to terminate the deposition process. Characterization The CNTs were characterized by SEM (JSM 7401F, 1.0 kV), high-resolution TEM (JEM 2010, 120.0 kV) and Raman spectroscopy (Horiba HR 800, 632.8 nm). An optical microscope (long working distance metallography microscope, FS-70Z) was used for the optical characterization and manipulation of individual CNTs. Cutting and transferring CNT segments The substrate with suspended CNTs was put on the stage of an optical microscope. Four probes were fixed on two pedestals on the microscope framework. The probes could be moved precisely in X, Y and Z directions by wheeling the knobs fixed on the pedestals. The four probes were taken into contact with the suspended CNTs, forming two scissor-like structures to cut the CNT. After a CNT segment was cut off, the probes then served as tweezers to transfer the CNT segment. Pulling out the inner tube from an individual DWCNT When the suspended DWCNTs decorated with TiO 2 NPs were placed under an optical microscope, the probes were taken into contact with the suspended DWCNTs. Then, the DWCNT was stretched by moving the probes in a certain direction. The deformation of the DWCNT could be directly monitored under the optical microscope. AFM cantilevers could be fixed onto the probes by silver paste to measure the forces applied on the DWCNTs. Gas-flow-induced bending of suspended CNTs A steady air flow was introduced through a glass tube (5 cm in length and 1 mm in diameter) to blow the suspended CNTs decorated with TiO 2 NPs. The fixed ends of the CNTs remained fixed when the suspended part was stretched. The elongation of the suspended CNTs was recorded by a digital camera (Carnon, SX500 IS). The gas velocity of the air flow was controlled by a mass flow metre (Sevenstar, CS200A 100SCC). Sound-wave-induced oscillation of suspended CNTs The suspended CNT/TiO 2 hybrids could be excited to oscillate by a sound wave from a loudspeaker linked to a signal generator (Tektronix, AFG3000C). The oscillation of the suspended CNTs was recorded by a digital camera (Carnon, SX500 IS). Manipulation of suspended CNTs in an electric field A minus voltage was applied on a suspended CNT, and a probe (with positive voltage) was used to attract the suspended CNT ( Supplementary Fig. S5a ). The suspended CNT is served as an electric field sensor and shows a quick response. Another example is shown in Supplementary Fig. S5b ; a 60-μm long free-drooping CNT was fixed on a metal probe with another probe placed 120 μm away. When a voltage was applied between the two probes (left: 2 V; right: −2 V), the suspended CNT was immediately attracted to the left probe ( Supplementary Fig. S5b (2)). Once the voltage was removed, the CNT immediately fell down back to a drooping state ( Supplementary Fig. S5b (3)). However, when an equal voltage was applied between the two probes (for example, 2 V for both probes), the strong electric repulsion between the two probes immediately repelled the freely drooping CNT away to the right side ( Supplementary Fig. S5b (4)). Once the voltage between the two probes was removed, the repelled CNT became drooping again. If the voltage difference between the two probes was applied again, the CNT would be immediately attracted to the left probe. Removing of the TiO 2 NPs from CNT A substrate with many TiO 2 NPs and short CNTs was put into a beaker containing 20 ml sulphuric acid solution (concentration 65%). (NH 4 ) 2 SO 4 powder of 8 g was added into the sulphuric acid solution as a dissolving promoter. Then the solution was heated to boil for 2 h. Then the substrate out was taken out and the TiO 2 NPs could be completely removed. How to cite this article: Zhang, R. et al . Optical visualization of individual ultralong carbon nanotubes by chemical vapour deposition of titanium dioxide nanoparticles. Nat. Commun. 4:1727 doi: 10.1038/ncomms2736 (2013).